Vasculogenic mimicry formation in EBV-associated epithelial malignancies 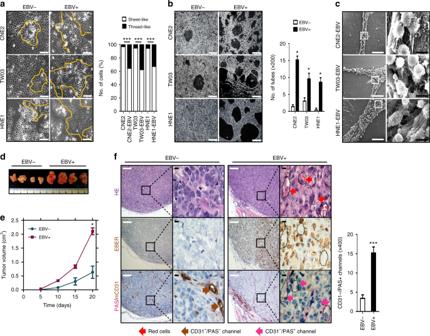Fig. 1 EBV infection promotes VM formation in vitro and in vivo.a(Left) Morphologies of EBV-infected NPC cells and their parental cells grown in conventional 2D culture plates. Cells are mixed with the sheet-like and thread-like cell types, and the latter were outlined with yellow lines. Scale bars = 100 μm. (Right) Quantification of the sheet-like and thread-like cell types in EBV-infected NPC cells and their parental cells. More than 100 cells were counted in randomly chosen fields. Mean ± SD,n= 5, ***p< 0.001 (two-tailed unpairedt-test).bImages (left) and quantification (right) of tube formation in EBV-infected NPC cells and their parental cells. Images were taken 12 h after seeding on Matrigel. Scale bars = 100 μm. Tubes were counted under a microscope with 200× magnification in randomly chosen fields. Mean ± SD,n= 5, *p< 0.05 (two-tailed Mann–Whitney test).cEBV-infected NPC cells displayed tubular networks and channels in 3D Matrigel, as observed by scanning electron microscopy. Scale bars = 100  μm (left panel), scale bars = 10 μm (right locally enlarged images).dCNE2 and CNE2-EBV cells were subcutaneously injected into nude mice, and images were taken 20 days post-implantation.eGrowth curves of xenograft tumors formed by CNE2 and CNE2-EBV cells. Mean ± SD,n=4, two-tailed Mann–Whitney test.fThe presence of VM in CNE2-EBV xenografts but not in control CNE2 xenografts. Pink arrows indicate VM channels (PAS+/mCD31−), which are formed by tumor cells (as stained by EBER) and containing red blood cells (stained by H&E; red arrows); brown arrows indicate typical blood vessels with brown mCD31+staining. White scale bars = 100 μm, black scale bars = 10 μm. (Left) Quantification of PAS+/mCD31−channels determined by microscopy with 400× magnification in randomly chosen fields. Mean ± SD,n= 5, ***p= 0.0002 (two-tailed unpairedt-test) Epstein-Barr virus (EBV)-associated epithelial cancers, including nasopharyngeal carcinoma (NPC) and approximately 10% of gastric cancers, termed EBVaGC, represent 80% of all EBV-related malignancies. However, the exact role of EBV in epithelial cancers remains elusive. Here, we report that EBV functions in vasculogenic mimicry (VM). Epithelial cancer cells infected with EBV develop tumor vascular networks that correlate with tumor growth, which is different from endothelial-derived angiogenic vessels and is VEGF-independent. Mechanistically, activation of the PI3K/AKT/mTOR/HIF-1α signaling cascade, which is partly mediated by LMP2A, is responsible for EBV-induced VM formation. Both xenografts and clinical samples of NPC and EBVaGC exhibit VM histologically, which are correlated with AKT and HIF-1α activation. Furthermore, although anti-VEGF monotherapy shows limited effects, potent synergistic antitumor activities are achieved by combination therapy with VEGF and HIF-1α-targeted agents. Our findings suggest that EBV creates plasticity in epithelial cells to express endothelial phenotype and provides a novel EBV-targeted antitumor strategy. Epstein-Barr virus (EBV) is a human cancer-associated virus that infects >90% of the global population. EBV infection is associated with a range of lymphoid and epithelial malignancies, such as Burkitt’s lymphoma, Hodgkin’s lymphoma, nasopharyngeal cancer (NPC), EBV-associated gastric cancer (EBVaGC), and others. For the past two decades, growing interest has focused on the EBV-associated epithelial cancers, which represent 80% of all EBV-associated malignancies. However, unlike the definitive role of EBV in the transformation of B lymphocytes to lymphoblastoid cell lines (LCLs), EBV infection does not lead to malignant transformation of normal epithelial cells, and interestingly, most primary NPC cells gradually lose EBV during passages in vitro, raising uncertainty about the causal role of EBV in the oncogenesis of epithelial cancers [1] . NPC and EBVaGC are the two most common EBV-associated epithelial cancers. NPC is a unique type of head and neck cancer arising from the nasopharynx and exhibiting a striking geographic and ethnic distribution, with unusually high incidence rates in southern China and South-East Asia. Almost 98% of all NPCs are EBV-associated [2] , [3] . In addition, ~10% of gastric carcinomas are associated with EBV (termed as EBVaGC) and represent a relatively non-endemic disease [4] , [5] . EBV infection is an early etiologic event in the evolution of NPC [6] . In most if not all NPC tumors, EBV displays type II latency, where EBV-encoded small RNA (EBER), EBV-associated nuclear antigen-1 (EBNA1), latent membrane protein 1/2 (LMP1 and LMP2), and BamHI A rightward transcript (BART)-microRNAs are expressed [3] , [7] , while EBV in EBVaGC is found to have latency I or II [5] . Although the transformation of premalignant epithelial cells into cancer cells by EBV remains controversial, EBV has been shown to have oncogenic properties, such as promoting cell growth, invasion, angiogenesis, and resistance to chemotherapy [3] , [8] , [9] . Defining the cellular processes targeted by EBV is crucial for understanding the role of EBV in tumor development and may provide effective therapeutic targets for EBV-associated diseases. It has been reported that the neoplastic disorders associated with EBV are related to enhanced angiogenesis [9] , [10] . Thus, anti-angiogenesis agents that target the vascular endothelial growth factor (VEGF) pathway are already in clinical trials of NPC [11] , [12] , [13] . While anti-VEGF therapy has achieved success in some solid tumors, failures in this approach due to inherent or acquired resistance have led to the urgent need to understand VEGF-independent angiogenesis [14] . In addition to classic angiogenesis, a new tumor vascular paradigm independent of endothelial cells (ECs), termed vasculogenic mimicry (VM), has emerged as another important vasculogenic mechanism in aggressive tumors. VM refers to the vascular channel-like structure that consists of tumor cells but not ECs. Periodic acid-Schiff (PAS) staining, hematoxylin and eosin (H&E) staining and CD31 immunohistochemistry (IHC) have been used to evaluate the presence of VM [15] , [16] . VM has been identified in various malignant tumors, including melanomas [15] , breast [17] , ovarian [18] , gastric [19] , lung [20] , and prostate cancers [21] . VM plays an essential role in the progression and metastasis of malignant tumors and actively participates in cancer growth, particularly under hypoxia [22] , [23] . In essence, VM is composed of cancer cells, and the mechanism of channel formation is different from vessels formed by ECs, thereby providing an explanation for the unsatisfactory response of VEGF-targeted therapy. To date, the presence of VM in NPC and EBVaGC and its relationship with EBV have not yet been demonstrated. In this study, we report a role for EBV in promoting VM formation in NPC and gastric cancer cells through the PI3K/AKT/mTOR/HIF-1α axis and demonstrate a potential application of HIF-1α as a therapeutic target for EBV-associated epithelial cancers that are resistant to anti-VEGF therapy. EBV infection promotes VM formation To investigate the role of EBV in epithelial cancers, we first established EBV-infected NPC cell lines as previously described [24] , [25] . Three typical NPC cell lines, CNE2, TW03, and HNE1, were infected with recombinant EBV derived from the Burkitt’s lymphoma cell line Akata-EBV. In situ hybridization confirmed the presence of EBER in the majority of cells in the EBV-infected cultures (Supplementary Fig. 1 ). Interestingly, EBV-negative and EBV-positive cell pairs displayed different morphologies: the parental EBV-negative NPC cells exhibited a cobblestone shape typical of epithelial cells, while the EBV-positive cells adopted an elongated spouting shape (Fig. 1a ). Next, we defined the growth patterns of these cells in 3D culture system. Strikingly, when seeded on a Matrigel surface, the EBV-positive cells formed loops and networks, while the EBV-negative cells spread evenly on the matrix surface (Fig. 1b ). To further define the structure of the tubular networks, scanning electron microscopy was performed on the 3D cultures. This approach confirmed that the structures formed by EBV+ NPC cells were indeed tubular and were lined externally with tumor cells (Fig. 1c ). The vessel-like structures resembled a phenomenon called VM, the process in which cancer cells form microvascular channels independent of angiogenesis [15] . To evaluate the VM formation in vivo, EBV− and EBV+ CNE2 cells were injected subcutaneously into nude mice. Twenty days post-implantation, the xenografts were dissected and examined for VM structures by double staining for the endothelial cell marker CD31 and periodic acid-Schiff (PAS), a reagent that detects polysaccharides outlining the basement membrane. The VM structure criteria were as follows: (1) vascular-like channels that were lined with EBER+ tumor cells; (2) positive for PAS but negative for CD31 (PAS + /CD31 − ); and (3) containing erythrocytes inside the channel, as demonstrated with H&E counterstaining (red arrows). Compared with the isogenic parental cells, CNE2 cells infected with EBV dramatically exacerbated tumor growth in the xenograft model (Fig. 1d, e ), and the tumors derived from EBV+ cells exhibited more VM structures (pink arrows) than those derived from EBV− NPC cells (Fig. 1f ), suggesting that EBV infection promotes the VM formation and tumorigenicity of NPC cells. Collectively, both the in vitro and in vivo data suggested that EBV plays an important role in VM. Fig. 1 EBV infection promotes VM formation in vitro and in vivo. a (Left) Morphologies of EBV-infected NPC cells and their parental cells grown in conventional 2D culture plates. Cells are mixed with the sheet-like and thread-like cell types, and the latter were outlined with yellow lines. Scale bars = 100 μm. (Right) Quantification of the sheet-like and thread-like cell types in EBV-infected NPC cells and their parental cells. More than 100 cells were counted in randomly chosen fields. Mean ± SD, n = 5, *** p < 0.001 (two-tailed unpaired t -test). b Images (left) and quantification (right) of tube formation in EBV-infected NPC cells and their parental cells. Images were taken 12 h after seeding on Matrigel. Scale bars = 100 μm. Tubes were counted under a microscope with 200× magnification in randomly chosen fields. Mean ± SD, n = 5, * p < 0.05 (two-tailed Mann–Whitney test). c EBV-infected NPC cells displayed tubular networks and channels in 3D Matrigel, as observed by scanning electron microscopy. Scale bars = 100  μm (left panel), scale bars = 10 μm (right locally enlarged images). d CNE2 and CNE2-EBV cells were subcutaneously injected into nude mice, and images were taken 20 days post-implantation. e Growth curves of xenograft tumors formed by CNE2 and CNE2-EBV cells. 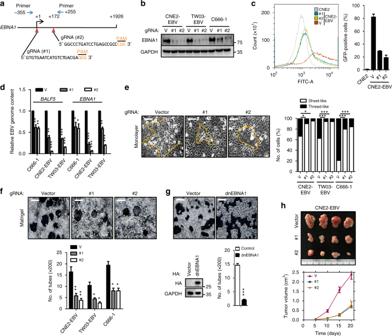Fig. 2 Clearance of EBV genomes reduces VM formation.aSchematic representation of theEBNA1gene and its gRNA target sites. Primers for T7E1 assay are shown (see Supplementary Fig.2a).bWestern blot analysis of EBNA1 in NPC-EBV cells transduced with control lentivirus or lentivirus expressing twoEBNA1gRNAs.cCNE2-EBV cells carrying recombinant EBV-GFP virions were subjected to CRISPR/Cas9-mediated EBV targeting as inb, and the GFP expression was determined by flow cytometry. Mean ± SD,n= 2.dRelative EBV copy numbers in NPC-EBV cells infected with control lentivirus or lentivirus carryingEBNA1gRNAs, as determined by real-time PCR using primers directed toBALF5andEBNA1. Data are represented as the mean ± SD,n= 3, two-tailed pairedt-test.e(left) Images of TW03-EBV cells transduced with control lentivirus or lentivirus expressingEBNA1gRNAs grown in conventional 2D culture plates. Scale bars = 100 μm. (right) Proportions of sheet-like and thread-like cell types were determined by microscopy with 200× magnification in randomly chosen fields. Mean ± SD,n= 5, two-tailed unpairedt-test with Welch’s correction.f(top) Images of the cells as ine, grown on 3D Matrigel. Scale bars = 50 μm. (bottom) Quantification of the tube numbers. Tubes were counted under a microscope with 200× magnification. Mean ± SD,n= 5, two-tailed Mann–Whitney test.gTube formation of CNE2-EBV cells transfected with empty vector or HA-tagged dominant-negative EBNA1 mutant (dnEBNA1). Mean ± SD,n= 5, two-tailed pairedt-test.h(top) Images of xenografts formed by CNE2-EBV cells transduced with lentiviral vector or lentivirus expressingEBNA1gRNA #1 or #2 at day 20 post-implantation. (bottom) Growth curves of xenografts formed by parental CNE2-EBV cells and CNE2-EBV cells subjected toEBNA1deletion by gRNA #1 and #2. Mean ± SD,n=4, two-tailed Mann–Whitney test. *p< 0.05, **p< 0.01 and ***p< 0.001 Mean ± SD, n = 4, two-tailed Mann–Whitney test. f The presence of VM in CNE2-EBV xenografts but not in control CNE2 xenografts. Pink arrows indicate VM channels (PAS + /mCD31 − ), which are formed by tumor cells (as stained by EBER) and containing red blood cells (stained by H&E; red arrows); brown arrows indicate typical blood vessels with brown mCD31 + staining. White scale bars = 100 μm, black scale bars = 10 μm. (Left) Quantification of PAS + /mCD31 − channels determined by microscopy with 400× magnification in randomly chosen fields. Mean ± SD, n = 5, *** p = 0.0002 (two-tailed unpaired t -test) Full size image Elimination of EBV decreases VM formation Next, we assessed the effects of the clearance of EBV genomes on VM formation. To this end, EBV nuclear antigen 1 (EBNA1), an essential gene for EBV maintenance and replication [26] , was deleted using CRISPR/Cas9 technology in two NPC cell lines (CNE2 and TW03) infected with Akata-derived EBV, and C666-1, the only NPC cell line containing the original-infecting EBV genome [27] . Two guide RNAs (gRNAs) targeting different regions of EBNA1 ending with a 5′NGG3′ protospacer-adjacent motif (PAM) sequence were used as described in a previous study [28] (Fig. 2a ). The editing efficiency of the gRNAs was confirmed by T7E1 assay (Supplementary Fig. 2a ), and the down-regulation of EBNA1 by the CRISPR/Cas9 system was demonstrated by Western blot analysis (Fig. 2b ). Next, the EBV genome content was analyzed. Upon transduction of EBNA1 gRNAs into CNE2 cells containing EBV-GFP virions, an ~60% reduction of GFP fluorescence was observed via flow cytometry (Fig. 2c and Supplementary Fig. 2b ) and fluorescence microscopy analyses (Supplementary Fig. 2c ). Furthermore, quantitative PCR with primers for the EBV BALF5 DNA polymerase gene also showed a significant reduction in EBV copy number in NPC-EBV cells following EBNA1 -deletion (Fig. 2d ), indicating that the viral genome had been successfully destructed by the CRISPR/Cas9 system. In line with the EBV infection data, clearance of EBV by CRISPR/Cas9 in NPC-EBV cells significantly decreased the percentage of cells displaying the elongated spouting shape (Fig. 2e ) and the number of tubes formed on Matrigel (Fig. 2f and Supplementary Fig. 2d ). In addition, using a dominant-negative mutant of EBNA1 (dnEBNA1) containing the DNA-binding/dimerization domain to compete against wild-type EBNA1 homodimers from binding to origin of replication ( oriP ) and thereby interrupting the maintenance of EBV episomes [29] , we showed that abrogation of EBNA1 activity had potent inhibitory effect on VM formation (Fig. 2g ). More importantly, EBNA1 deletion led to a decreased tumor burden and decelerated tumor growth over time (Fig. 2h ) compared with those of the parental cells with intact EBV genome. Collectively, these results indicated that the VM formation of NPC cells depends on the existence of EBV. Fig. 2 Clearance of EBV genomes reduces VM formation. a Schematic representation of the EBNA1 gene and its gRNA target sites. Primers for T7E1 assay are shown (see Supplementary Fig. 2a ). b Western blot analysis of EBNA1 in NPC-EBV cells transduced with control lentivirus or lentivirus expressing two EBNA1 gRNAs. c CNE2-EBV cells carrying recombinant EBV-GFP virions were subjected to CRISPR/Cas9-mediated EBV targeting as in b , and the GFP expression was determined by flow cytometry. Mean ± SD, n = 2. d Relative EBV copy numbers in NPC-EBV cells infected with control lentivirus or lentivirus carrying EBNA1 gRNAs, as determined by real-time PCR using primers directed to BALF5 and EBNA1 . Data are represented as the mean ± SD, n = 3, two-tailed paired t -test. e (left) Images of TW03-EBV cells transduced with control lentivirus or lentivirus expressing EBNA1 gRNAs grown in conventional 2D culture plates. Scale bars = 100 μm. (right) Proportions of sheet-like and thread-like cell types were determined by microscopy with 200× magnification in randomly chosen fields. Mean ± SD, n = 5, two-tailed unpaired t -test with Welch’s correction. f (top) Images of the cells as in e , grown on 3D Matrigel. Scale bars = 50 μm. (bottom) Quantification of the tube numbers. Tubes were counted under a microscope with 200× magnification. Mean ± SD, n = 5, two-tailed Mann–Whitney test. g Tube formation of CNE2-EBV cells transfected with empty vector or HA-tagged dominant-negative EBNA1 mutant (dnEBNA1). Mean ± SD, n = 5, two-tailed paired t -test. h (top) Images of xenografts formed by CNE2-EBV cells transduced with lentiviral vector or lentivirus expressing EBNA1 gRNA #1 or #2 at day 20 post-implantation. (bottom) Growth curves of xenografts formed by parental CNE2-EBV cells and CNE2-EBV cells subjected to EBNA1 deletion by gRNA #1 and #2. Mean ± SD, n = 4, two-tailed Mann–Whitney test. * p < 0.05, ** p < 0.01 and *** p < 0.001 Full size image Transcriptome analysis reveals hallmarks of VM in NPC-EBV To gain mechanistic insights into VM formation by EBV infection, we compared global gene expression profiles of the paired EBV-positive and EBV-negative cells (CNE2-EBV vs. CNE2 and TW03-EBV vs. TW03) using RNA-seq analysis. In total, 4644 and 3634 differentially expressed genes (DEGs) (fold change ≥ 2) were found in CNE2 and TW03 cell pairs, respectively (Fig. 3a ). Functional profiling of the 1399 overlapping DEGs suggested that the affected genes were enriched in biological processes including PI3K-AKT pathway, proteoglycans in cancer, TNF signaling pathways and others (Fig. 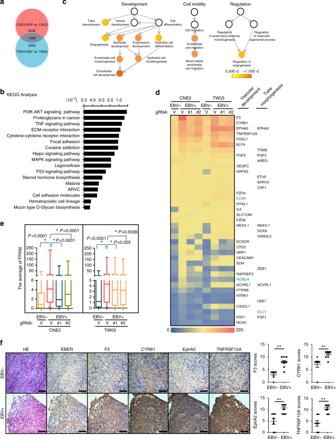Fig. 3 Enrichment of VM-related genes by EBV infection.aVenn diagram illustrating the overlap of differentially expressed genes (DEGs) in paired EBV-negative and EBV-positive NPC cells (CNE2 vs. CNE2-EBV and TW03 vs. TW03-EBV) by RNA-seq.bBar plot ranking of the top enrichment score (p-value) values for the significant enrichment pathways according to KEGG analysis of DEGs between EBV− and EBV+ NPC cells. Only pathways withp< 0.05 are shown.cGO tree obtained from BiNGO showing the hierarchy of biological processes related to endothelial cell development, endothelial cell migration and angiogenesis between the EBV-positive and EBV-negative NPC cell pairs (padj< 0.05; see the color bar). The white nodes (padj> 0.05) were added to show the relationships among their downstream nodes.dHeatmap depicting FPKM values for vascular development and tube morphogenesis-related genes in EBV− and EBV+ NPC cell pairs and EBV+ cells withEBNA1deletion by gRNAs.padj< 0.05. Of note, 36 out of 39 of these genes contain HRE motif in their promoter region (Supplementary Fig.3) with the exception of three genes colored in green.eThe average FPKM values of the DEGs ind. ns: not significant (one-tailed Wilcoxon matched pairs test).f(left) Serial sections of EBV-negative and EBV-positive NPC tissues were stained with H&E, EBER and antibodies targeting F3, CYR61, EphA2 and TNFRSF12A. Scale bars = 500 μm. (right) IHC scores of the indicated genes in 10 EBV-positive and 7 EBV-negative NPC biopsies. Means ± SD, **p< 0.01, two-tailed Mann–Whitney test 3b ). Importantly, Gene Ontology (GO) function classification showed that processes including endothelial cell development, endothelial cell migrations and angiogenesis-related genes were differentially expressed in EBV-negative and EBV-positive NPC cell pairs, indicating that EBV infection might change the expression of VM-related genes (Fig. 3c ). Therefore, we focused on the DEGs that were associated with neovascularization, including vascular development and tube morphogenesis. A total of 39 genes in these groups were consistently up-regulated in the two EBV-positive cell lines compared with their EBV-negative counterparts and after EBV genome destruction (Fig. 3d, e ). The upregulation of these genes were further confirmed by IHC staining in NPC samples. Using 10 EBV-positive and 7 EBV-negative NPC biopsies (see Methods for detailed sample information), we showed that some DEGs in Fig. 3d , including F3, CYR61, EphA2, and TNFRSF12A, were indeed upregulated in EBV-positive NPC samples (Fig. 3f ). The above analysis indicated that the 39 vasculogenesis-related genes may account for EBV-induced VM formation. Fig. 3 Enrichment of VM-related genes by EBV infection. a Venn diagram illustrating the overlap of differentially expressed genes (DEGs) in paired EBV-negative and EBV-positive NPC cells (CNE2 vs. CNE2-EBV and TW03 vs. TW03-EBV) by RNA-seq. b Bar plot ranking of the top enrichment score ( p -value) values for the significant enrichment pathways according to KEGG analysis of DEGs between EBV− and EBV+ NPC cells. Only pathways with p < 0.05 are shown. c GO tree obtained from BiNGO showing the hierarchy of biological processes related to endothelial cell development, endothelial cell migration and angiogenesis between the EBV-positive and EBV-negative NPC cell pairs ( p adj < 0.05; see the color bar). The white nodes ( p adj > 0.05) were added to show the relationships among their downstream nodes. d Heatmap depicting FPKM values for vascular development and tube morphogenesis-related genes in EBV− and EBV+ NPC cell pairs and EBV+ cells with EBNA1 deletion by gRNAs. p adj < 0.05. Of note, 36 out of 39 of these genes contain HRE motif in their promoter region (Supplementary Fig. 3 ) with the exception of three genes colored in green. e The average FPKM values of the DEGs in d . ns: not significant (one-tailed Wilcoxon matched pairs test). f (left) Serial sections of EBV-negative and EBV-positive NPC tissues were stained with H&E, EBER and antibodies targeting F3, CYR61, EphA2 and TNFRSF12A. Scale bars = 500 μm. (right) IHC scores of the indicated genes in 10 EBV-positive and 7 EBV-negative NPC biopsies. Means ± SD, ** p < 0.01, two-tailed Mann–Whitney test Full size image HIF-1α is required for EBV-induced VM formation To investigate the regulatory mode of the aforementioned vasculogenesis-related genes upregulated by EBV infection, a search for promoter modules of these genes was conducted. Strikingly, promoters for 36 out of 39 vasculogenesis-related genes were found to harbor the HIF-1-response element (HRE) consensus sequence 5′-RCGTG-3′ [30] (Supplementary Fig. 3 ). HIF-1 is a heterodimeric transcription factor consisting of an oxygen-sensitive subunit HIF-1α and a constitutively expressed HIF-1β subunit, which plays a critical role in VM formation [22] , [31] , [32] . Under normoxia, HIF-1α is located in the cytoplasm and is targeted for von Hippel Lindau (VHL)-mediated rapid destruction by proline hydroxylation. Under hypoxic conditions, HIF-1α prolyl hydroxylation is decreased, causing the dissociation of HIF-1α with VHL complex in the cytoplasm, thus enabling HIF-1α stabilization and nuclear accumulation to heterodimerize with HIF-1β. The HIF complex then binds to HRE on target genes and activates their transcription, which functions to increase oxygen delivery [33] . We then analyzed HIF-1α expression in the paired EBV-negative and EBV-positive NPC cells. Real-time PCR showed that HIF-1α mRNA levels were similar in EBV− and EBV+ NPC cell pairs (Supplementary Fig. 4a ). We then examined the protein levels and subcellular localization of HIF-1α. Immunofluorescence showed a dim cytoplasmic staining of HIF-1α in EBV-negative NPC cells; in contrast, strong nuclear staining of HIF-1α was observed in EBV-positive NPC cells. Conversely, deletion of EBNA1 by gRNAs in NPC-EBV cells abrogated the nuclear accumulation of HIF-1α (Fig. 4a, b and Supplementary Fig. 4b ). Similarly, a subcellular fractionation assay also demonstrated the nuclear accumulation of HIF-1α following EBV infection (Fig. 4c ). Next, we investigated the role of HIF-1α in EBV-induced VM formation. Using HIF-1α inhibitor PX-478 to suppress HIF-1α expression (Fig. 4d, e and Supplementary Fig. 4c , top panel), we showed that the in vitro VM formation of NPC-EBV cells was severely impaired by HIF-1α inhibition (Supplementary Fig. 4c , bottom panel) in a dose-dependent manner (Fig. 4f and Supplementary Fig. 4d ), while the cell viability was not affected below the concentration of 10 μM (Supplementary Fig. 4e ). Similar observations were obtained by using 2MeOE2, another HIF-1α inhibitor that blocks HIF-1α accumulation and activity [34] (Fig. 4g, h ). Furthermore, knockdown of HIF-1α with specific siRNAs severally impaired VM formation of EBV-infected cells (Fig. 4i, j ). These data indicate that EBV-induced HIF-1α activation contributes to VM formation. Fig. 4 EBV-induced VM formation is HIF-1α-dependent. a Immunofluorescence of HIF-1α in TW03 and TW03-EBV cells with or without targeting of EBV by CRISPR/Cas9. Scale bars = 50 μm. b The mean integrated optical density (MOD) values of HIF-1α levels in the cytoplasm and nucleus of NPC cells with or without EBV. More than 100 cells were counted in randomly chosen fields. Mean ± SD, n = 3, two-tailed unpaired t -test. c Subcellular fractionation of EBV- cells, EBV+ cells and EBV+ cells subjected to EBV targeting by transfecting EBNA1 gRNAs. Each extract was analyzed by immunoblotting of HIF-1α, β-Tubulin, and PARP1. β-Tubulin represents cytoplasmic proteins, and PARP1 is used as a nuclear protein marker. d EBV− and EBV+ NPC cells were treated with 10 or 50 μM PX-478 for 24 h, followed by WB analysis of HIF-1α. e Immunofluorescence staining of HIF-1α in TW03-EBV cells that were treated with 10 μM PX-478 for 24 h or left untreated. Scale bars = 50 μm. f (left) Light microscopy of the tube formation of TW03-EBV cells that were pre-treated with 10 μM PX-478 for 24 h prior to plating on Matrigel for additional 12 h. Scale bars = 100 μm. (right) Quantification of the tube numbers formed by NPC-EBV cells after PX-478 treatment at different concentrations, as indicated. Mean ± SD, n = 5, two-tailed unpaired t -test. g EBV- and EBV+ TW03 cells were treated with 1 or 10 μM 2-MeOE2 for 12 h, followed by WB analysis of HIF-1α. h (left) In vitro tube formation of TW03-EBV cells that were treated with DMSO or 10 μM 2-MeOE2 for 12 h on Matrigel. Scale bars = 100 μm. (right) Quantification of tube numbers formed by NPC-EBV cells after 2-MeOE2 treatment. Mean ± SD, n = 5, two-tailed Mann–Whitney test. i Immunoblotting of NPC cells transfected with control or HIF-1α-specific siRNAs. j (left) Images and (right) quantification of tube formation of control and HIF-1α-depleted cells. Scale bars = 100 μm. Mean ± SD, n = 5, two-tailed Mann–Whitney test. ns: not significant, * p < 0.05, ** p < 0.01 and *** p < 0.001 Full size image EBV increases HIF-1α synthesis via PI3K-AKT-mTOR pathway In addition to hypoxia, pathways involved in oncogenic activation also activate HIF-1α in an oxygen-independent manner, such as loss of PTEN and VHL and gain-of-function mutations in oncogenes in PI3K-AKT-mTOR and MAPK pathways [35] , [36] . Among these molecules, PI3K-AKT pathway is the most significantly affected pathway in EBV-infected NPC cells (Fig. 3b ). As expected, EBV infection led to an increase in AKT phosphorylation; conversely, elimination of EBV through the CRISPR/Cas9 system reduced AKT phosphorylation to levels similar to that of the EBV-negative control cells (Fig. 5a, b and Supplementary Fig. 5a ). The effect of EBV targeting was specific to EBV-positive cells, as transduction of EBNA-1 gRNAs into EBV-negative NPC cells had no effects on the levels of phospho-AKT and HIF-1α (Supplementary Fig. 5b ). Additionally, transfection of dominant-negative mutant of EBNA-1 into EBV-positive cells resulted in a marked suppression of AKT phosphorylation and HIF-1α expression (Fig. 5c ). We then treated EBV+ cells with LY294002 and Wortmannin, two inhibitors of PI3K. Both drugs effectively reduced total (Fig. 5d ) and nuclear HIF-1α accumulation to levels similar to those of the EBV-negative counterparts under normoxic conditions (Fig. 5e, f and Supplementary Fig. 5c , top panel). Furthermore, LY294002 and Wortmannin suppressed the in vitro VM formation of EBV-infected NPC cells (Fig. 5g and Supplementary Fig. 5c , bottom panel) in a dose-dependent manner (Fig. 5h and Supplementary Fig. 5d ), indicating the involvement of PI3K-AKT signaling in EBV-induced HIF-1α accumulation and VM formation. Fig. 5 EBV promotes VM formation via the PI3K/AKT/mTOR/HIF-1α axis. a Immunofluorescence of phospho-AKT (S473) in TW03 cells and TW03-EBV cells with or without targeting EBV by CRISPR/Cas9. Scale bars = 50 μm. b Immunoblots comparing AKT phosphorylation in EBV- and EBV+ NPC cell lines. c CNE2-EBV cells were transfected with empty vector or a dominant-negative mutant of EBNA1 (dnEBNA1), followed by WB analysis using antibodies as indicated. d Immunoblots of AKT phosphorylation and HIF-1α expression following LY294002 (50 μM) or Wortmannin (1 μM) treatment for 6 h. e Immunoblots of HIF-1α distribution in cytoplasmic and nuclear fractions of EBV- and EBV+ NPC cells following LY294002 (50 μM), Wortmannin (1 μM) or DMSO treatment for 6 h. f Immunofluorescence of phospho-AKT (S473) and HIF-1α in TW03-EBV cells after 6 h of treatment with DMSO, LY294002 (50 μM) or Wortmannin (1 μM). Scale bars = 50 μm. g Microscopy of tube formation on Matrigel in TW03-EBV cells after 12 h of treatment with LY294002 (50 μM) or Wortmannin (1 μM). Scale bars = 100 μm. h Quantification of tube numbers formed by NPC-EBV cells following LY294002 or Wortmannin treatment. Mean ± SD, n = 5, two-tailed unpaired t -test. i Effects of PI3K/mTOR/S6K kinase inhibitors on EBV-induced HIF-1α expression. CNE2-EBV cells were treated with DMSO, 1 μM Wortmannin (Wort), 0.5 μM rapamycin (Rapa) or 10 μM PF-4708671 (PF) for 6 h under normoxic conditions prior to immunoblotting with antibodies, as indicated. j Effect of rapamycin (0.5 μM) on VM channel formation of CNE2-EBV cells. Mean ± SD, n = 5, two-tailed unpaired t -test. ns: not significant, * p < 0.05, *** p < 0.001 Full size image AKT affects multiple downstream targets. One of the downstream protein kinases, mTOR (mammalian target of rapamycin), has been implicated in PI3K/AKT-dependent oncogenesis through its regulation of cap-dependent translation initiation by phosphorylating two downstream effectors, eukaryotic initiation factor 4E (eIF4E)-binding protein (4E-BP1) and p70 S6 kinase (S6K) [37] , [38] . Notably, it has been shown that the mTOR pathway increases HIF-1α translation driven by the 5’ UTR region of HIF-1α [39] . We then treated CNE2-EBV cells with the mTOR inhibitor rapamycin and the S6K inhibitor PF-4708671 to delineate the mTOR pathway in EBV-induced HIF-1α. The accumulation of HIF-1α in EBV-infected cells was highly sensitive to mTOR and S6K inhibitors to a similar extent as with the PI3K inhibitor Wortmannin, while the expression of the EBV immediate-early gene Zta was not affected by these drugs (Fig. 5i ). The capacity of PF-4708671 to inhibit mTOR phosphorylation might be due to the direct phosphorylation of mTOR by S6K [40] . Correspondingly, rapamycin significantly inhibited VM network formation of CNE2-EBV cells (Fig. 5j ). We also compared the degradation rate of HIF-1α in EBV-negative and EBV-positive CNE2 cells and the results suggested that the presence of EBV did not decelerate HIF-1α degradation; besides, HIF-1α hydroxylation, which is required for the interaction with VHL E3 ubiquitin ligase, was not inhibited by EBV infection, suggesting that EBV does not contribute to HIF-1α stabilization (Supplementary Fig. 5e ). Together, these results indicate that EBV promotes VM formation through PI3K/AKT/mTOR-mediated HIF-1α synthesis. LMP2A regulates VM formation through the AKT/HIF-1α axis Having established the role of EBV in promoting VM, we next tried to identify the viral genes that contribute to VM formation. As EBV typically exists in latency, we first examined the latent gene expression patterns in EBV-infected NPC cell lines. RT-PCR results suggested that EBNA1 , LMP1 , and LMP2A were all expressed in CNE2-EBV, HNE1-EBV, and C666-1 cells, while LMP2B transcript was absent in C666-1 cells as described previously [27] ; on the contrary, the transcription of latency III antigen EBNA2 was only detected in the B-cell line, B95-8 (Fig. 6a ), therefore the expression pattern of EBV-infected NPC cells corresponded to type II latency, the same as in NPC tumors. Among these latent genes, LMP1 and LMP2A have been implicated in AKT activation. However, given that LMP1 is detected in only 10–20% of NPCs by immunohistostaining [8] and could not be detected by Western blots of C666-1 cells [27] , and as LMP1 is often absent in EBVaGC [4] , [5] , we focused on LMP2A, an EBV oncoprotein constitutively activates AKT [41] , [42] and mTOR pathways [43] and is more consistent in NPC [7] . As expected, overexpression of LMP2A in NPC cells (CNE2 and HNE1) led to increases in the levels of phosphorylated AKT, mTOR, 4E-BP1, S6K and ribosomal protein S6, accompanied by upregulation of HIF-1α (Fig. 6b ). Furthermore, NPC cells overexpressing LMP2A readily formed tubes on Matrigel, which was not evident in cells transfected with empty vector (Fig. 6c ). More importantly, knockdown of LMP2A with siRNA reduced HIF-1α expression and PI3K/AKT/mTOR signaling axis activation (Fig. 6d ), as well as the tube-forming capacities of EBV-infected NPC cells (Fig. 6e ), supporting an important role for LMP2A in EBV-induced VM formation. Fig. 6 LMP2A is involved in VM formation and AKT/HIF-1α activation. a RT-PCR analysis of EBV latent genes in CNE2 and HNE1 cells carrying recombinant EBV (Akata strain) and the native EBV-infected cell line C666-1. GAPDH was used as the internal control. b CNE2 and HNE1 cells were transfected with empty vector or construct encoding LMP2A. Activation of AKT/mTOR/HIF-1α signaling pathway was determined by immunoblotting. c Representative images (top) and quantification (bottom) of tube formation on Matrigel of control and LMP2A-overexpressing NPC cells. Scale bars = 100 μm. Tube numbers were counted under a microscope with 200× magnification in randomly chosen fields. Mean ± SD, n = 5, two-tailed Mann–Whitney test. d CNE2-EBV and TW03-EBV cells were transfected with control or LMP2A-specific siRNAs. The knockdown efficiency was determined by RT-PCR, and HIF-1α level and AKT/mTOR/S6K signaling activity were determined by immunoblotting. e Representative images (left) and quantification (right) of tube formation of NPC-EBV cells transfected with control or LMP2A-specific siRNA. Scale bars = 100 μm. Mean ± SD, n = 5, two-tailed Mann–Whitney test. ** p < 0.01 and *** p < 0.001 Full size image EBV links to VM formation in EBV-associated carcinomas Next, we investigated the correlation between AKT/HIF-1α activity and VM formation in xenografts and human NPC and gastric carcinoma tissues. Xenografts derived from EBV-infected CNE2 cells showed increased AKT phosphorylation, HIF-1α nuclear accumulation and VM structure compared with EBV-negative CNE2-derived tumors (Supplementary Fig. 6a ). We further investigated VM formation in human NPC tissues. The VM channels positive for PAS and negative for CD31 (pink arrows) were lined with EBER-positive tumor cells and contained red blood cells (Fig. 7a , top panel). Quantification of IHC staining results demonstrated that the PAS + CD31 − NPC tumor cells expressed high levels of EBER, phospho-AKT, and HIF-1α (Fig. 7b ). These data confirmed the existence of VM in NPC clinical samples and further demonstrated the association between EBV infection, VM formation, and AKT/HIF-1α activation. Fig. 7 Correlation of VM with EBV infection in NPC and EBVaGC. a (top) NPC and (bottom) EBV-negative and EBV-positive gastric carcinoma serial sections were stained with H&E, EBER, PAS, and antibodies targeting human CD31, p-AKT, and HIF-1α. White scale bars = 100 μm, black scale bars = 10 μm. b Pearson correlation of PAS + /CD31 − tumor cells of VM with EBER, phosphorylated AKT or nuclear HIF-1α staining in NPC tissue. p < 0.001, r = regression coefficient. c Pearson correlation of PAS + /CD31 − tumor cells with the staining as in b in EBV− and EBV+ human gastric carcinoma samples, p < 0.001 Full size image To determine whether the effect of EBV on VM formation was limited to NPC or also applied to other EBV-associated tumors, we examined VM formation in EBV− and EBV+ gastric carcinomas, the latter of which is known as EBV-associated gastric carcinoma (EBVaGC). An in vitro VM assay using a pair of EBV− and EBV+ gastric carcinoma cell lines, AGS and AGS-EBV, along with two EBV-positive gastric carcinoma cell lines, GT38 and GT39, demonstrated that EBV-positive gastric carcinoma cells formed tubes on 3D Matrigel culture, which did not occur in the EBV-negative AGS cells (Supplementary Fig. 6b, c ). More importantly, histological analysis of human gastric carcinoma tissues suggested that EBVaGC displayed more VM structures and expressed higher levels of phospho-AKT and nuclear HIF-1α than did EBV-negative gastric carcinoma tissue (Fig. 7a , bottom panel and c), indicating that EBV plays a general role in VM formation via the AKT/HIF-1α axis in EBV-associated epithelial malignancies. Synergistic effect of anti-VM and anti-VEGF therapy in NPC VEGF is a key tumor angiogenesis factor and is regulated by HIF-1α. As EBV infection led to HIF-1α accumulation, we next investigated the involvement of VEGF in EBV-induced VM formation. Indeed, EBV infection increased VEGF secretion (Supplementary Fig. 7a ). However, blocking autocrine VEGF by anti-human VEGF neutralization antibody (NAb) did not have an appreciable effect on the tube formation of EBV-infected NPC cells; in contrast, a strong inhibition of the tube formation of human umbilical vein endothelial cells (HUVECs) was observed following VEGF NAb treatment (Supplementary Fig. 7b ). Additionally, treatment of EBV-positive NPC cells with Axitinib, a selective inhibitor of VEGF receptors, did not affect in vitro VM formation (Supplementary Fig. 7c ), indicating that VEGF did not contribute to the EBV-induced VM. Based on the above findings, we proposed that concurrent targeting of VEGF-mediated classic angiogenesis and VM might achieve maximal antitumor efficacy in EBV-associated tumors. Therefore, we evaluated the effects of anti-VEGF or anti-HIF-1α monotherapy and combination therapy in NPC xenografts. Treatment with the HIF-1α inhibitor PX-478 or the VEGFR inhibitor Axitinib alone only showed modest anti-tumor effects. In contrast, combination of PX-478 and Axitinib induced a significantly more pronounced tumor inhibition (Fig. 8a, b ). We then assessed tumor neovascularization by histological double staining of CD31 and PAS. Tumors from the control group were enriched in both ECs and VM channel-like structures, and treatment with Axitinib decreased CD31 + microvessels (brown) without affecting VM formation (PAS + /CD31 − , pink), whereas PX-478 treatment led to large areas of VM loss without a significant reduction in microvessels. Notably, the combination of Axitinib and PX-478 caused marked decreases in both microvessels and VM (Fig. 8c–e ). These results suggest that targeting VEGF and HIF-1α has synergistic anti-angiogenic effects, providing a novel therapeutic option for EBV-associated tumors. Fig. 8 Synergistic effects of PX-478 and Axitinib in NPC-EBV. a Image of CNE2-EBV xenograft tumors from mice treated with vehicle, Axitinib alone (30 mg kg −1 p.o., twice a day), PX-478 (5 mg kg −1 p.o., every 2 days) alone or Axitinib plus PX-478. b Growth curves of CNE2-EBV xenograft tumors after treatment with vehicle, Axitinib or/and PX-478. Mean ± SD, n = 10, *** p < 0.001 versus the other three treatment groups (two-tailed Mann–Whitney test). c H&E, PAS and mouse CD31 staining of CNE2-EBV xenograft sections. Red lines: necrotic area. White scale bars = 100 μm, black scale bars = 50 μm. d Numbers of endothelial cell (EC) channel-like structures in CNE2-EBV xenograft tumors from mice treated with vehicle, Axitinib or/and PX-478. Channels were determined under a microscope with 400× magnification in randomly chosen fields. Mean ± SD, n = 5, two-tailed Mann–Whitney test. e Number of VM channel-like structures in CNE2-EBV xenografts counted as in d . f Working model illustrating the mechanism by which EBV promotes VM and the aggressiveness of carcinomas such as NPC and EBVaGC. ns: not significant, * p < 0.05, *** p < 0.001 Full size image EBV was the first human DNA tumor virus discovered over 50 years ago [1] . EBV has been linked to the development of cancers originating from both lymphoid and epithelial cells. However, the contribution of the virus to epithelial cell tumors is less clear. but is generally believed to be a consequence of the aberrant establishment of virus latency in epithelial cells that undergo premalignant genetic changes [3] , [7] . Although EBV infection may not be the initiating event for epithelial cell tumors, EBV has been shown to change the host gene expression profile and signaling networks to endow cancerous properties, including increased cell survival, proliferation, invasion, angiogenesis, immune evasion, EMT, and acquisition of stemness features [3] , [8] , [9] , [44] , [45] . In this study, we show that EBV infection confers neovascular features in epithelial cancers by promoting VM formation. Cells infected with EBV readily form an extensive network of tube-like structures in vitro that is reminiscent of endothelial blood vessels; furthermore, VM structures, as defined by PAS + /CD31 − staining, were evident in NPC and EBVaGC biopsies. Our finding that epithelial cells infected with EBV phenotypically mimic endothelial-like cells further indicates that EBV creates plasticity in host cells. It is widely accepted that tumors require blood supply for growth; these vasculogenic-like networks induced by the virus could serve as an intratumoral fluid-conducting meshwork to contribute to the growth advantage of EBV-infected tumors. EBV infection leads to the epigenetic changes, involving DNA methylation and histone modifications, and signaling pathway aberrations in host cells [8] , [46] . Our transcriptome analysis revealed that vasculogenesis-related genes were upregulated in EBV-infected epithelial cells. Interestingly, the promoters of most of these genes contain the HRE motif (Supplementary Fig. 3 ). HIF-1α is constitutively stabilized in normoxic EBV-associated tumors, and inhibition of HIF-1α by PX-473 suppressed the VM phenotype and xenograft tumor progression, highlighting the importance of HIF-1α in VM formation and the optimal growth of EBV-associated tumors. The relationship between EBV latent genes and HIF-1α is complex. For example, LMP1 has been shown to enhance HIF-1α synthesis through ERK1/2 MAPK signaling [47] ; LMP1 has also been demonstrated to stabilize HIF-1α through down-regulation of prolyl hydroxylases [48] . In addition, EBNA1 promotes HIF-1α transcription in NPC cells [49] , and EBNA3A stabilizes HIF-1α via binding to prolyl hydroxylases in B lymphocytes [50] . However, these above-mentioned studies were mostly performed by overexpressing of a single EBV gene, which could not fully recapitulate the biological phenotype of natural EBV infection. In this study, we established isogenic EBV-negative and EBV-positive NPC cells and demonstrated that the PI3K/AKT pathway, the most significantly perturbed pathway following EBV infection, mediates primarily non-hypoxic HIF-1α regulation in EBV-infected epithelial cells. 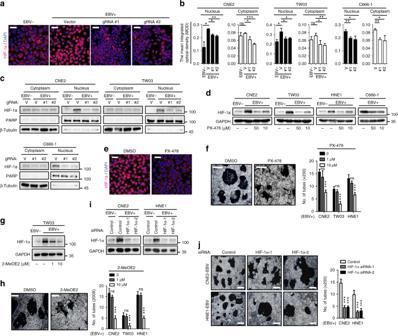Fig. 4 EBV-induced VM formation is HIF-1α-dependent.aImmunofluorescence of HIF-1α in TW03 and TW03-EBV cells with or without targeting of EBV by CRISPR/Cas9. Scale bars = 50 μm.bThe mean integrated optical density (MOD) values of HIF-1α levels in the cytoplasm and nucleus of NPC cells with or without EBV. More than 100 cells were counted in randomly chosen fields. Mean ± SD,n= 3, two-tailed unpairedt-test.cSubcellular fractionation of EBV- cells, EBV+ cells and EBV+ cells subjected to EBV targeting by transfectingEBNA1gRNAs. Each extract was analyzed by immunoblotting of HIF-1α, β-Tubulin, and PARP1. β-Tubulin represents cytoplasmic proteins, and PARP1 is used as a nuclear protein marker.dEBV− and EBV+ NPC cells were treated with 10 or 50 μM PX-478 for 24 h, followed by WB analysis of HIF-1α.eImmunofluorescence staining of HIF-1α in TW03-EBV cells that were treated with 10 μM PX-478 for 24 h or left untreated. Scale bars = 50 μm.f(left) Light microscopy of the tube formation of TW03-EBV cells that were pre-treated with 10 μM PX-478 for 24 h prior to plating on Matrigel for additional 12 h. Scale bars = 100 μm. (right) Quantification of the tube numbers formed by NPC-EBV cells after PX-478 treatment at different concentrations, as indicated. Mean ± SD,n= 5, two-tailed unpairedt-test.gEBV- and EBV+ TW03 cells were treated with 1 or 10 μM 2-MeOE2 for 12 h, followed by WB analysis of HIF-1α.h(left) In vitro tube formation of TW03-EBV cells that were treated with DMSO or 10 μM 2-MeOE2 for 12 h on Matrigel. Scale bars = 100 μm. (right) Quantification of tube numbers formed by NPC-EBV cells after 2-MeOE2 treatment. Mean ± SD,n= 5, two-tailed Mann–Whitney test.iImmunoblotting of NPC cells transfected with control or HIF-1α-specific siRNAs.j(left) Images and (right) quantification of tube formation of control and HIF-1α-depleted cells. Scale bars = 100 μm. Mean ± SD,n= 5, two-tailed Mann–Whitney test. ns: not significant, *p< 0.05, **p< 0.01 and ***p< 0.001 Mechanistically, EBV drives HIF-1α synthesis through PI3K-AKT-mTOR-mediated protein translation, but plays little roles in HIF-1α transcription and protein degradation (Supplementary Fig 4a , 5e ). mTOR is a key downstream mediator in the PI3K/AKT signaling pathway that plays a central role in regulating cap-dependent translation of HIF-1α [39] . Among latent proteins, both LMP1 and LMP2A contribute to AKT [8] , [41] , [42] and mTOR activation [43] , [51] . However, LMP1 expression is variable in NPC and is often absent in EBVaGC [4] , [5] , and it has been shown that LMP1 is not associated with HIF-1α expression in NPC tissues [52] . On the contrary, LMP2A expression is consistently detected in various EBV-associated malignancies, pointing out its essential role in pathogenesis. LMP2A is an integral membrane protein whose amino terminus recruits tyrosine kinases Lyn and Syk to activate PI3K-AKT signaling [8] . We demonstrated that LMP2A is required for PI3K/AKT/mTOR/HIF-1α cascade activation and the VM formation driven by EBV (Fig. 8f ). Whether LMP2A coordinates with other EBV genes/miRNAs to orchestrate HIF-1α expression and VM formation needs further investigation. On the other side, VM might be attributable to the maintenance of viral latency as the tumor enlarges. Latent infection is known to be necessary for virus persistence and immune evasion. Solid tumors develop regions of hypoxia when they outgrow their blood supply, and it has been demonstrated that hypoxia reactivates EBV to lytic replication through binding to the HRE motif on the promoter of the immediate-early BZLF1/Zta gene [53] , [54] . As reported, ectopically expression of wild-type and consitutively active (CA) mutant of HIF-1α [55] upregulated Zta mRNA level and protein abundance, and hypoxia-stabilized HIF-1α protein to drive Zta transcription (Supplementary Fig. 8a–c ). Our study revealed that VM induced by EBV infection is associated with HIF-1α activation. However, abrogation of HIF-1α accumulation by pharmacological targeting PI3K/AKT/mTOR pathway, or by depletion of LMP2A in EBV-infected cells, did not lead to reduction in Zta level (Figs. 5h and 6d ), indicating that the extent of non-hypoxic HIF-1α upregulation driven by EBV does not reach the threshold for virus lytic activation as hypoxia does. Establishment of a greater oxygen delivery capacity while maintaining long-term persistent viral infection may be the physiological significance of VM formation and is a survival strategy of EBV, which could be a required step in the progression of EBV-associated carcinomas. Our results suggest that VM status should be taken into account for anti-angiogenic therapy in patients with EBV-associated epithelial cancers. Angiogenesis has been considered as a promising treatment target in NPC. Bevacizumab, a chimeric monoclonal antibody targeting VEGF, has been evaluated in a Phase II multinational trial in combination with standard chemoradiation treatment in 46 NPC patients [13] . Another tyrosine kinase inhibitor targeting VEGF receptor, sunitinib, has been tested in a Phase II study in 13 metastatic NPC patients [12] . However, these studies have been discontinued because of severe hemorrhagic events, even though patients showed tumor shrinkage. Furthermore, VEGF inhibition may cause a hypoxic and acidic microenvironment, which accelerates tumor progression [56] . Therefore, targeting alternative neovascularization pathways might be a logical way to overcome the resistance to anti-VEGF therapy. Our approach to use combination therapy with Axitinib and PX-478 provides a means to circumvent the development of resistance to conventional antiangiogenesis therapy, and the finding of the role of HIF-1α in EBV-induced VM opens a new avenue to further explore the clinical use of HIF-1α inhibitors in NPC and EBVaGC. In addition to HIF-1, targeting additional stages in VM signaling, such as inhibition of mTOR pathway using rapamycin analogs, would achieve similar therapeutic effects. Further studies of the molecular pathways that regulate EBV-induced VM formation could lead to new strategies to target EBV-associated epithelial cancers and could provide new perspectives on EBV-induced tumor cell plasticity. Cell culture Akata-EBV-GFP is an Akata Burkitt lymphoma cell line carrying the Akata bacterial artificial chromosome (BAC) with a GFP tag, B95-8 is an EBV-producing marmoset B-cell line, both were cultured in RPMI 1640 medium with 10% fetal bovine serum (FBS) (Hyclone). The NPC cell lines CNE2, HNE1, TW03, and C666-1 were cultured in RPMI-1640 with 5% FBS. B cell lines and NPC cell lines were from Prof. Mu-Sheng Zeng (Sun Yat-sen University Cancer Center). The gastric carcinoma cell lines AGS, AGS-EBV, GT38, and GT39 were kindly provided by Prof. Rui-Hua Xu (Sun Yat-sen University Cancer Center) and cultured in DMEM (Hyclone) with 5% FBS. All cell lines were routinely tested and shown to be Mycoplasma-free as determined by PCR-based method (16S rDNA-F: 5′-ACTCCTACGGGAGGCAGCAGTA-3′, 16S rDNA-R: 5′-TGCACCATCTGTCACTCTGTTAACCTC-3′). Establishment of EBV-infected cells For EBV production, Akata-EBV-GFP cells were treated with 0.8% (v/v) goat anti-human IgG for 6 h to induce EBV transition from the latent phase into the lytic cycle. After culture in fresh medium for 3 days, the supernatants were collected by centrifugation at 20,000× g for 30 min at 4 ℃. The pellets were resuspended in 10% FBS DMEM and used for cell-free infection. The infected CNE2, HNE1, TW03, and AGS cells were sorted using flow cytometry (Beckman) and were maintained in culture medium containing 300–700 μg mL −1 G418 (Invitrogen). The infection was verified by in situ hybridization (ISH) of EBER according to the manufacturer’s instructions for the EBER ISH kit (Zhongshan Jinqiao Bio. Co.). Western blot analysis Cells were lysed in SDS-loading buffer, the lysates were resolved on SDS–PAGE and transferred to PVDF membrane (Millipore). The blots were then incubated with species-specific HRP-conjugated secondary antibodies, and the immunoreactive bands were visualized by enhanced chemiluminescence (ECL, Pierce). Full Western blot images are shown in Supplementary Fig. 9 . Antibodies, chemicals, and siRNAs The following antibodies were used in this study: mouse monoclonal HIF-1α antibody (sc-13515, Santa Cruz. 1:50 for IF), rabbit monoclonal HIF-1α antibody (ab51608, Abcam. 1:100 for IHC, 1:500 for WB), Hydroxy-HIF-1α (Pro564) (3434, Cell Signaling Technology. 1:1000 for WB), phospho-AKT (Ser473) (4060, Cell Signaling Technology. 1:100 for IF, 1:1000 for WB), phospho-AKT (Ser473) (ab81283, Abcam. 1:100 for IHC), AKT (9272, Cell Signaling Technology. 1:2000 for WB), phospho-mTOR (Ser2448) (2971, Cell Signaling Technology, 1:1000 for WB), mTOR (2983, Cell Signaling Technology. 1:2000 for WB), phospho-S6K (Thr389) (9205, Cell Signaling Technology, 1:1000 for WB), S6K (2708, Cell Signaling Technology, 1:1000 for WB), phospho-4E-BP1 (Thr37/46) (2855, Cell Signaling Technology, 1:1000 for WB), phospho-S6 (Ser235/236) (2211, Cell Signaling Technology. 1:1000 for WB), ribosomal protein S6 (2317, Cell Signaling Technology, 1:500 for WB), anti-mouse CD31 antibody (77699, Cell Signaling Technology. 1:100 for IHC), anti-human CD31 antibody (3528, Cell Signaling Technology, 1:100 for IHC), EBNA1 (ab81581, Abcam, 1:500 for WB), LMP2A (ab59028, Abcam. 1:500 for WB and only recognizes the overexpressed protein), F3 (ab104513, Abcam, 1:50 for IHC), CYR61 (ab10760, Abcam, 1:200 for IHC), EphA2 (ab5386, Abcam, 1:100 for IHC) and TNFRSF12A (ab109365, Abcam, 1:100 for IHC), PARP (9542, Cell Signaling Technology, 1:2000 for WB), Zta/ZEBRA (sc-53904, Santa Cruz, 1:200 for WB), GAPDH (60004-1-1g, Protein-tech, 1:5000 for WB), β-Tubulin (2128, Cell Signaling Technology, 1:2000 for WB), and VEGF (AB-293-NA, R&D Systems. 1 μg mL −1 for neutralization). Horseradish peroxidase-conjugated goat anti-mouse/rabbit secondary antibodies were purchased from Promega. PX-478, LY294002, Wortmannin, 2-Methoxyestradiol (2-MeOE2), and Axitinib were purchased from Selleckchem. SiRNAs were synthesized by Guangzhou RiboBio Co., Ltd., and the sequences were as follows: Control siRNA: 5′-UUCAAUAAAUUCUUGAGGUdTdT-3′; siRNA targeting Akata LMP2A: 5′-CUGGCAUACUCUUCAUUCUdTdT-3′. siRNA targeting HIF-1a: #1: 5′-UGCUCUUUGUGGUUGGAUCUA-3′, #2: 5′-CCGCUGGAGACACAAUCAUAU-3′. Lipofectamine RNAiMAX (Invitrogen) was used for siRNA transfection. Constructs and CRISPR/Cas9-mediated EBNA1 deletion LMP2A cDNA of Akata strain was subcloned into the pCDH vector. A dnEBNA1 (consists of NLS aa 379–386 and the C-terminal DNA linking/dimerization domain aa 451–641) [29] was subcloned to the pCDH vector with a HA tag at the C terminus. CRISPR/Cas9 genome-editing system was used to delete EBV EBNA1 [25] , [28] . Two gRNAs targeting EBNA1 , gRNA#1: 5′-GTGTGAATCATGTCTGACGA-3′ and gRNA#2:5′-GGCCCTGATCCTGAGCCGCC-3′, were cloned into the lentiviral transfer vector Lenti-CRISPRv2 and were used to package lentiviral particles. For lentiviral packaging, lentiviral vector was co-transfected with the packaging plasmids pMD2.G and psPAX2 into HEK293T cells; 48 h post-transfection, the supernatant was collected and used for infection. Stable EBNA1 -deleted cells were selected with 2 μg mL −1 puromycin. The EBV clearance effect was assessed by detecting EBV genome content by real-time PCR of the BALF5 gene and by counting the percentage of GFP-expressing cells using flow cytometry and fluorescence microscopy. Real-time PCR and semi-quantitative RT-PCR Total RNA was isolated with TRIzol reagent (Invitrogen) according to the manufacturer’s instructions. First-strand cDNA was synthesized using a PrimeScript RT Reagent Kit (TaKaRa). The EBV genome content was determined by real-time PCR analysis of the BALF5 gene with primers as follows: BALF5 -F: 5′-CGGAGTTGTTATCAAAGAGGC-3′, BALF5 -R: 5′-CGAGAAAGACGGAGATGGC-3′. Detection of EBV-encoded transcripts was performed by semi-quantitative RT-PCR using gene specific primers as follows: EBNA1 -F: 5′-GGACCCGGCCCACAACCTG-3′, EBNA1 -R: 5′- CTACTCCCACTCCTTCCCGTCCTC-3′; LMP1 -F:5′- GCGACTCTGCTGGAAATGAT -3′, LMP1 -R: 5′- GACATGGTAATGCCTAGAAG -3′; LMP2A -F: 5′-ATGACTCATCTCAACACATA-3′, LMP2A -R: 5′-CATGTTAGGCAAATTGCAAA-3′; LMP2B -F: 5′- CAGTGTAATCTGCACAAAGA-3′, LMP2B -R: 5′- CATGTTAGGCAAATTGCAAA-3′; EBNA2 -F: 5′- AGAGGAGGTGGTAAGCGGTTC-3′, EBNA2 -R: 5′- TGACGGGTTTCCAAGACTATCC-3′; GAPDH -F: 5′-GGTGGTCTCCTCTGACTTCAACA-3′, GAPDH -R: 5′-GTTGCTGTAGCCAAATTCGTTGT-3′. Animal studies All of the animal experiments were approved by the Institutional Animal Care and Use Committee of Sun Yat-sen University (reference no. L102042016110W), and the animals were handled in accordance with institutional guidelines. Female BALB/c nude mice (4–6 weeks old) purchased from Shanghai Laboratory Animal Center were inoculated subcutaneously in the right flanks with 5 × 10 6 CNE2 and CNE2-EBV cells. Tumor volume ( V ) was measured by caliper every 2 days for the duration of the experiment and calculated with the formula V = (length × width 2 )/2. For antitumor drug assessment, when tumors reached 100–200 mm 3 , the mice were randomized divided into four groups ( n = 10 for each group). The control group received vehicle (0.5% sodium carboxymethyl cellulose (CMC)) daily, and the treatment groups received either Axitinib (30 mg kg −1 p.o., twice daily) alone, PX-478 (5 mg kg −1 p.o., every two days) alone or a combination of Axitinib and PX-478. 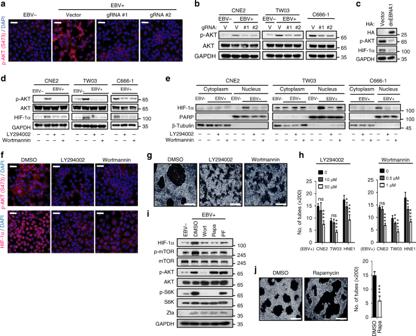Fig. 5 EBV promotes VM formation via the PI3K/AKT/mTOR/HIF-1α axis.aImmunofluorescence of phospho-AKT (S473) in TW03 cells and TW03-EBV cells with or without targeting EBV by CRISPR/Cas9. Scale bars = 50 μm.bImmunoblots comparing AKT phosphorylation in EBV- and EBV+ NPC cell lines.cCNE2-EBV cells were transfected with empty vector or a dominant-negative mutant of EBNA1 (dnEBNA1), followed by WB analysis using antibodies as indicated.dImmunoblots of AKT phosphorylation and HIF-1α expression following LY294002 (50 μM) or Wortmannin (1 μM) treatment for 6 h.eImmunoblots of HIF-1α distribution in cytoplasmic and nuclear fractions of EBV- and EBV+ NPC cells following LY294002 (50 μM), Wortmannin (1 μM) or DMSO treatment for 6 h.fImmunofluorescence of phospho-AKT (S473) and HIF-1α in TW03-EBV cells after 6 h of treatment with DMSO, LY294002 (50 μM) or Wortmannin (1 μM). Scale bars = 50 μm.gMicroscopy of tube formation on Matrigel in TW03-EBV cells after 12 h of treatment with LY294002 (50 μM) or Wortmannin (1 μM). Scale bars = 100 μm.hQuantification of tube numbers formed by NPC-EBV cells following LY294002 or Wortmannin treatment. Mean ± SD,n= 5, two-tailed unpairedt-test.iEffects of PI3K/mTOR/S6K kinase inhibitors on EBV-induced HIF-1α expression. CNE2-EBV cells were treated with DMSO, 1 μM Wortmannin (Wort), 0.5 μM rapamycin (Rapa) or 10 μM PF-4708671 (PF) for 6 h under normoxic conditions prior to immunoblotting with antibodies, as indicated.jEffect of rapamycin (0.5 μM) on VM channel formation of CNE2-EBV cells. Mean ± SD,n= 5, two-tailed unpairedt-test. ns: not significant, *p< 0.05, ***p< 0.001 Tumor sizes were measured every other day. At the end of the experiment, mice were euthanized, and tumors were harvested and weighed. In vitro tube formation assay Briefly, 30 μL of Matrigel (BD) was plated in 96-well plates and incubated at 37 °C for 30 min to allow polymerization. Next, 1 × 10 5 cells per well were added to the Matrigel layer and grown for 12 h. Randomized fields were captured using an inverted microscope, and tubes were quantified from each image. Data are presented as the average number of tubes ± SD. Scanning electron microscopy For scanning electron microscopy, EBV-positive NPC cells were added to the Matrigel-treated coverslips for 12 h and then fixed in 2.5% cold glutaraldehyde in 0.1 M of sodium cacodylate buffer (pH 7.4). Specimens were dehydrated in a graded series of ethanol, transferred in acetone and isoamyl acetate and then subjected to critical point drying with CO 2 in a HITACHI HCP-2. Dried samples were sputter-coated with gold with a Giko IB.5 ion coater before scanning electron microscopy (FEI QUANTA 200, 20 kV) observation. Clinical specimens Clinical sample collection from human patients was approved by the Human Research Ethics Committee of the Sun Yat-sen University cancer center (GZR2016-105), and written informed consent was obtained from all participants. In total, 10 cases EBV-positive (seven males and three females from ages 42 to 61, all are primary NPC tumors) and seven cases EBV-negative NPCs (five males and two females from ages 35 to 70, including one case of primary tumor and six cases of recurrent tumors), five cases of EBV-positive (five males from ages 33 to 53) and seven cases of EBV-negative human gastric carcinoma (four males and three females from ages 48 to 84) were obtained from Sun Yat-sen University cancer center, Guangzhou, China, from 2010 to 2017, and all of the samples were diagnosed by two pathologists (Dr. Jinping Yuan and Dr. Jianyong Shao, Sun Yat-sen University Cancer Center). Ten cases of EBV-positive NPC tumors, one case of primary EBV-negative NPC tumor and human gastric carcinomas had not received anti-tumor treatment before biopsy collection; six cases of recurrent EBV-negative NPCs received intensity modulated radiation therapy(IMRT) with or without platinum-based concurrent chemotherapy. IHC and PAS staining IHC was performed on formalin-fixed paraffin-embedded (FFPE) sections of clinical NPC and gastric cancer tissues or xenograft mice tissues. Briefly, the tissues were deparaffinized and rehydrated, and the samples were subjected to citrate-mediated high-temperature antigen retrieval and the samples were incubated with the primary antibodies at 4 °C overnight [57] . 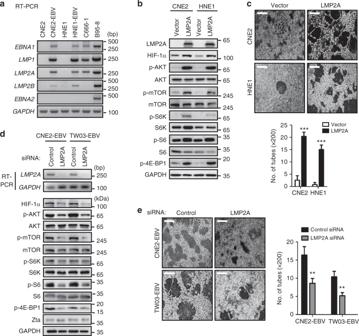Fig. 6 LMP2A is involved in VM formation and AKT/HIF-1α activation.aRT-PCR analysis of EBV latent genes in CNE2 and HNE1 cells carrying recombinant EBV (Akata strain) and the native EBV-infected cell line C666-1. GAPDH was used as the internal control.bCNE2 and HNE1 cells were transfected with empty vector or construct encoding LMP2A. Activation of AKT/mTOR/HIF-1α signaling pathway was determined by immunoblotting.cRepresentative images (top) and quantification (bottom) of tube formation on Matrigel of control and LMP2A-overexpressing NPC cells. Scale bars = 100 μm. Tube numbers were counted under a microscope with 200× magnification in randomly chosen fields. Mean ± SD,n= 5, two-tailed Mann–Whitney test.dCNE2-EBV and TW03-EBV cells were transfected with control or LMP2A-specific siRNAs. The knockdown efficiency was determined by RT-PCR, and HIF-1α level and AKT/mTOR/S6K signaling activity were determined by immunoblotting.eRepresentative images (left) and quantification (right) of tube formation of NPC-EBV cells transfected with control or LMP2A-specific siRNA. Scale bars = 100 μm. Mean ± SD,n= 5, two-tailed Mann–Whitney test. **p< 0.01 and ***p< 0.001 A semiquantitative scoring was evaluated as follows: 0 for staining in ≤ 1% of cancer cells, 1 for staining in 2–25% of cancer cells, 2 for staining in 26–50% of cancer cells, 3 for staining in 51–75% of cancer cells, and 4 for staining in ≥ 75% of cancer cells. Staining intensity was scored as 0, no staining; 1, weak staining; 2, moderate staining; and 3, strong staining. Staining was repeated at least twice in sequential sections from the same tissue blocks, and the sections were reviewed by two pathologists. The staining index (values 0–12) was obtained by multiplying the intensity by the proportion of immunopositive cells of interest. To detect VM structures, a PAS staining kit (BASO BA-4080A) was applied before hematoxylin counterstaining. the numbers of positive cells were counted from ≥ 5 randomly chosen fields. Whole-transcriptome sequencing Total RNA was isolated with TRIzol and purified using the RNeasy Plus Micro Kit (Qiagen) according to the manufacturer’s protocol. The RNA libraries were then sequenced using the Illumina HiSeq4000 at the Novogene Genomic Sequencing Center, Beijing, China. The RNA-seq sequence reads were aligned to the reference genome using STAR (v2.5.1b). Differential expression analysis was performed using the DESeq2 R package (1.10.1). The resulting P -values were adjusted using the Benjamini and Hochberg’s approach for controlling the false discovery rate. Genes with an adjusted p -value ( p adj ) < 0.05 and an absolute fold change of 2 were set as the threshold for significantly differential expression. The alignment results were converted to RNA-seq gene expression measurements as FPKM (fragments per kilobase of exon per million fragments mapped) using HTSeq v0.6.0. Immunofluorescence and nuclear/cytosol fractionation Cells were seeded on coverslips and fixed with 4% paraformaldehyde. After washing with PBS, coverslips were incubated with 0.2% Triton X-100 for 5 min. Cells were incubated with the primary antibodies for 1 h and then with Alexa Fluor 594 goat anti-mouse or goat anti-rabbit IgG (Invitrogen) for 1 h. Cells were then counterstained with DAPI (Sigma) and imaged with a confocal laser-scanning microscope (Olympus FV1000) [57] . To quantify the Immunofluorescence intensity, the integrated optical density (IOD) was calculated using Image J software, and the mean IOD (MOD) was calculated from IOD/Area. 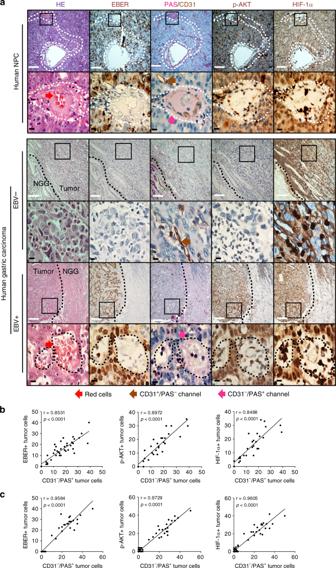Fig. 7 Correlation of VM with EBV infection in NPC and EBVaGC.a(top) NPC and (bottom) EBV-negative and EBV-positive gastric carcinoma serial sections were stained with H&E, EBER, PAS, and antibodies targeting human CD31, p-AKT, and HIF-1α. White scale bars = 100 μm, black scale bars = 10 μm.bPearson correlation of PAS+/CD31−tumor cells of VM with EBER, phosphorylated AKT or nuclear HIF-1α staining in NPC tissue.p< 0.001,r= regression coefficient.cPearson correlation of PAS+/CD31−tumor cells with the staining as inbin EBV− and EBV+ human gastric carcinoma samples,p< 0.001 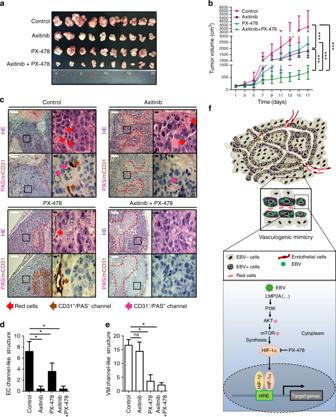Fig. 8 Synergistic effects of PX-478 and Axitinib in NPC-EBV.aImage of CNE2-EBV xenograft tumors from mice treated with vehicle, Axitinib alone (30 mg kg−1p.o., twice a day), PX-478 (5 mg kg−1p.o., every 2 days) alone or Axitinib plus PX-478.bGrowth curves of CNE2-EBV xenograft tumors after treatment with vehicle, Axitinib or/and PX-478. Mean ± SD,n= 10, ***p< 0.001 versus the other three treatment groups (two-tailed Mann–Whitney test).cH&E, PAS and mouse CD31 staining of CNE2-EBV xenograft sections. Red lines: necrotic area. White scale bars = 100 μm, black scale bars = 50 μm.dNumbers of endothelial cell (EC) channel-like structures in CNE2-EBV xenograft tumors from mice treated with vehicle, Axitinib or/and PX-478. Channels were determined under a microscope with 400× magnification in randomly chosen fields. Mean ± SD,n= 5, two-tailed Mann–Whitney test.eNumber of VM channel-like structures in CNE2-EBV xenografts counted as ind.fWorking model illustrating the mechanism by which EBV promotes VM and the aggressiveness of carcinomas such as NPC and EBVaGC. ns: not significant, *p< 0.05, ***p< 0.001 Nuclear/cytosol fractionation was performed using the Nuclear-Cytosol Extraction Kit (KeyGen, Nanjing, China) according to the manufacturer’s instructions. Statistical analysis Unless otherwise stated, data with a Gaussian distribution were compared with a two-tailed unpaired t -test or a two-tailed unpaired t -test with Welch’s correction if variances were significantly different, as determined by the F-test. Matched samples with a Gaussian distribution were compared with a two-tailed paired t -test. Matched samples with non-Gaussian distribution were compared with a Wilcoxon matched pairs test. Data with a non-Gaussian distribution were compared with a two-tailed Mann–Whitney test. Pearson’s correlation coefficient was used to determine the correlations of VM with EBER, AKT phosphorylation and nuclear HIF-1α expression.